The tumour suppressorLKB1regulates myelination through mitochondrial metabolism A prerequisite to myelination of peripheral axons by Schwann cells (SCs) is SC differentiation, and recent evidence indicates that reprogramming from a glycolytic to oxidative metabolism occurs during cellular differentiation. Whether this reprogramming is essential for SC differentiation, and the genes that regulate this critical metabolic transition are unknown. Here we show that the tumour suppressor Lkb1 is essential for this metabolic transition and myelination of peripheral axons. Hypomyelination in the Lkb1 -mutant nerves and muscle atrophy lead to hindlimb dysfunction and peripheral neuropathy. Lkb1 -null SCs failed to optimally activate mitochondrial oxidative metabolism during differentiation. This deficit was caused by Lkb1 -regulated diminished production of the mitochondrial Krebs cycle substrate citrate, a precursor to cellular lipids. Consequently, myelin lipids were reduced in Lkb1 -mutant mice. Restoring citrate partially rescued Lkb1 -mutant SC defects. Thus, Lkb1 -mediated metabolic shift during SC differentiation increases mitochondrial metabolism and lipogenesis, necessary for normal myelination. Mitochondrial metabolic dysfunctions are a common cause of numerous neurodegenerative disorders and are important contributors to peripheral neuropathy. Much is known about the neuronal metabolic changes that cause neuropathy [1] . However, the mechanisms by which peripheral nerve glial (Schwann cell) metabolism contributes to disease pathology are only being recently elucidated in SC-specific mitochondrial dysfunction studies [2] , [3] . This dearth of knowledge is despite the facts that SCs provide crucial long-term functional support to peripheral axons [4] , [5] and abnormal mitochondria in the nerves of neuropathy patients have often been localized to SCs [6] , [7] . SCs ensheath axons in the peripheral nervous system (PNS), wrapping around axons and assembling myelin. Myelination increases axonal membrane resistance and reduces capacitance allowing high-velocity salutatory conduction of electrical impulses. In mice, shortly after birth, neural crest-derived SCs stop proliferation, differentiate and start assembling myelin. Peripheral myelination is essentially complete for the most part within the first 3 weeks of life. Although much is known about SC transcriptional programs and axonal signals that regulate myelination, it is unclear if other SC-intrinsic changes are needed for optimal SC differentiation and myelination. In light of the increasing appreciation that proliferating cells undergo considerable metabolic reprogramming during differentiation [8] , [9] , [10] , [11] , [12] , we tested the hypothesis that a shift to mitochondrial metabolism is required for optimal myelination, and metabolic genes regulate this process. The tumour suppressor Lkb1/STK11 is a metabolic kinase crucial for embryonic development [13] , [14] . It regulates cellular functions including growth, survival, migration, polarity, mitochondrial respiration and cell differentiation [15] , [16] , [17] , [18] , [19] . To directly interrogate whether Lkb1 function is required for metabolic reprogramming and myelination, we generated myelinating glia-specific Lkb1 -knockout mice (henceforth Lkb1 -mutant mice). We report that proliferating SCs undergo metabolic reprogramming from glycolytic to oxidative metabolism during differentiation and myelination in vivo and in vitro , and that Lkb1 is essential for this metabolic shift. Our findings show that hypomyelination is due to a deficit in the production of the tricarboxylic acid (TCA) cycle metabolite citrate, a precursor to cellular lipids. Mitochondrial deficits in Lkb1 -mutant SCs and sciatic nerve are also echoed by reduced mitochondrial oxygen consumption and membrane potential. Collectively, our study suggests that metabolic reprogramming occurs in SCs, which is a required step during myelination, and a cell-intrinsic defect in mitochondrial metabolism regulated by Lkb1 causes hypomyelination and neuropathy in Lkb1 -mutant mice. Lkb1 -mutant mice have peripheral neuropathy To directly examine the function of the metabolic kinase Lkb1 in SC biology, we generated myelin-forming glial cell-specific Lkb1 -knockout mice by crossing Lkb1 lox/lox or lox/− ( Fig. 1a ; Supplementary Fig. 1a ) [13] mice with Cnp-Cre knock-in mice [20] . CNP (2′,3′-cyclic nucleotide 3′-phosphodiesterase) is highly expressed in myelin-forming glial cells and Cre expression driven by the Cnp1 regulatory elements is widely used to examine function of genes in these glial cells. To confirm that Cre expression is restricted to glia, we crossed Cnp-Cre mice with CAG-CAT-EGFP-floxed reporter mice [21] . Green fluorescent protein (GFP) expression was evident in sciatic nerves ( Fig. 1b ), brain ( Supplementary Fig. 1b )and both GFP and Cre expression co-localized to SCIP (OCT6) + SCs of sciatic nerves ( Supplementary Fig. 1c ). GFP expression was excluded from NeuN + neurons in the brain ( Supplementary Fig. 1d ). Western blot analysis of cultured dorsal root ganglia (DRG) neurons and purified SCs showed Lkb1 protein in Lkb1 lox/lox;Cre DRG neurons but not in SCs ( Fig. 1c ). Immunofluorescence analysis also showed Lkb1 loss in SCIP + SCs in the sciatic nerves of Lkb1 lox/−;cre mice ( Supplementary Fig. 1e ). Axonal neurofilament expression was unchanged in these mice ( Supplementary Fig. 1f ). Together, these results confirm that Cre-mediated recombination resulted in Lkb1 loss in SCs but not in neurons. 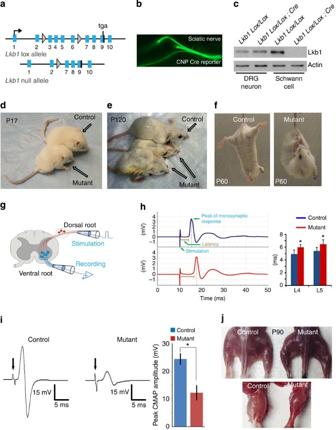Figure 1:Lkb1-mutant mice demonstrate peripheral neuropathy and motor abnormalities. (a) Conditional mutagenesis ofLkb1-floxed gene that eliminates exons 3–6 causing a translational frameshift. (SeeSupplementary Fig. 1Afor genotyping PCR and methods for breeding strategy). (b) Enhanced GFP fluorescence in sciatic nerve of mice derived from matings betweenCnp-Cremice andCAG-CAT-EGFP loxreporter mice demonstratingCreexpression in the PNS. (c) Western blot analysis showing loss of Lkb1 protein in SCs but not in DRG neurons. Actin was used as a protein loading control. Data are representative of two independent experiments. (d) Growth retardation in youngLkb1-mutant mice. (e) Severe emaciation and kyphosis (hunchback) of 4-month-oldLkb1-mutant mice. (f) When lifted by the tail, adultLkb1-mutant mice but not WT (control) mice demonstrated hindlimb clasping. Cartoon (g) of genotype-blinded extracellular recordings (h) of L4 and L5 ventral roots from control (upper, blue) andLkb1-mutant (lower, red) mice. Dotted lines show the peak of monosynaptic response. Inset shows the average of latency of monosynaptic responses from control (blue) andLkb1-mutant (red) mice (n=3 control and 3 mutant P6 mice). Error bars show s.d. (*P≤0.02). Data are representative of two independent experiments. (i) CMAP recordings in 2-month-old control andLkb1-mutant mice. Inset shows significant reduction in the peak CMAP amplitude inLkb1-mutant mice compared with controls (n=3 control and 3 mutant mice). Arrows indicate onset of electrical stimulation of the sciatic nerve during recording. Error bars show s.d. (*P=0.002). Data are representative of two independent experiments. (j) Representative images showing hindlimb muscle atrophy inLkb1-mutant mice (upper panel: entire hindlimb; lower panel: gastrocnemius muscle). Student’st-test was used to calculate statistical significance. Figure 1: Lkb1 -mutant mice demonstrate peripheral neuropathy and motor abnormalities. ( a ) Conditional mutagenesis of Lkb1 -floxed gene that eliminates exons 3–6 causing a translational frameshift. (See Supplementary Fig. 1A for genotyping PCR and methods for breeding strategy). ( b ) Enhanced GFP fluorescence in sciatic nerve of mice derived from matings between Cnp-Cre mice and CAG-CAT-EGFP lox reporter mice demonstrating Cre expression in the PNS. ( c ) Western blot analysis showing loss of Lkb1 protein in SCs but not in DRG neurons. Actin was used as a protein loading control. Data are representative of two independent experiments. ( d ) Growth retardation in young Lkb1 -mutant mice. ( e ) Severe emaciation and kyphosis (hunchback) of 4-month-old Lkb1 -mutant mice. ( f ) When lifted by the tail, adult Lkb1 -mutant mice but not WT (control) mice demonstrated hindlimb clasping. Cartoon ( g ) of genotype-blinded extracellular recordings ( h ) of L4 and L5 ventral roots from control (upper, blue) and Lkb1 -mutant (lower, red) mice. Dotted lines show the peak of monosynaptic response. Inset shows the average of latency of monosynaptic responses from control (blue) and Lkb1 -mutant (red) mice ( n =3 control and 3 mutant P6 mice). Error bars show s.d. (* P ≤0.02). Data are representative of two independent experiments. ( i ) CMAP recordings in 2-month-old control and Lkb1 -mutant mice. Inset shows significant reduction in the peak CMAP amplitude in Lkb1 -mutant mice compared with controls ( n =3 control and 3 mutant mice). Arrows indicate onset of electrical stimulation of the sciatic nerve during recording. Error bars show s.d. (* P =0.002). Data are representative of two independent experiments. ( j ) Representative images showing hindlimb muscle atrophy in Lkb1 -mutant mice (upper panel: entire hindlimb; lower panel: gastrocnemius muscle). Student’s t -test was used to calculate statistical significance. Full size image Lkb1 -mutant animals were born at expected Mendelian ratios and were indistinguishable from littermates at birth and until the end of the first week of life. By postnatal day 14 (P14), the mutant animals showed growth retardation (likely due to reduced ability to compete for milk; Fig. 1d ), but no visible signs of neuropathy (for example, trembling/shaking) or reduction in brain size ( Supplementary Fig. 1g ) were observed. By P30, mutant adult animals showed difficulty in supporting their body weight on their hindlimbs ( Supplementary Fig. 2a ) and died prematurely if food was not left inside the cage. By 4 months, about 50% of mutant animals were emaciated ( Fig. 1e ) and required euthanasia. The mutant animals demonstrated abnormal gait ( Supplementary Fig. 2b ; Supplementary Movie 1a,b ), hindlimb clasping when lifted by the tail ( Fig. 1f ), and were unable to grasp a horizontal cylinder with their hindlimbs ( Supplementary Fig. 2c ; Supplementary Movie 2a,b ). A battery of locomotion and behavioural tests ( Supplementary Fig. 2d ; Supplementary Movie 3 ) indicated peripheral nerve disease as reported in other mouse models of peripheral neuropathy [22] , [23] , [24] . Since Lkb1 -mutant animals showed hindlimb dysfunction, we first examined sensory-motor connections in P5–P7 mice. Monosynaptic latency was longer in Lkb1 mutants compared with wild-type (WT) mice ( Fig. 1g,h ), suggestive of possible myelination defects. Myelination defects could cause neuromuscular conduction deficits, which is a possible cause of muscle atrophy and hindlimb dysfunction as seen in many human peripheral neuropathies. We therefore examined nerve conduction in adult mice. Compound muscle action potentials (CMAPs) were obtained from the lateral gastrocnemius muscle during electrical stimulation of the sciatic nerve in vivo . Peak CMAP amplitude was significantly decreased in Lkb1 -mutant mice compared with control animals ( Fig. 1i ). Not surprisingly, this profound defect in nerve conduction correlated with and is the likely cause of significant hindlimb muscle atrophy ( Fig. 1j ). Together, these findings show that Lkb1 loss in SCs causes significant hindlimb dysfunction, muscle weakness and loss of body weight support by hindlimbs. Lkb1 -mutant mice have hypomyelination in the PNS The hindlimb dysfunctions of the Lkb1 -mutant mice prompted us to interrogate the state of myelination in these mice. At P10 (when myelination in the mouse PNS is robust), sciatic nerves of Lkb1 -mutant mice were thinner and less opaque than control nerves ( Supplementary Fig. 2e ), indicative of reduced myelination. Toluidine blue staining of semithin plastic sections of P30 sciatic nerves showed global hypomyelination in the Lkb1 -mutant sciatic nerve ( Supplementary Fig. 2f,g ). Electron microscopic (EM) examination of sciatic nerves at P30 confirmed that >90% of axons were hypomyelinated in the Lkb1 -mutant sciatic nerve ( Fig. 2a–c ) with rare (~4.5%) unmyelinated or severely hypomyelinated axons ( Supplementary Fig. 3a ). In myelinated axons, G-ratio analysis (the ratio between the diameter of the axon and the total fibre (axon+myelin sheath)) demonstrated a significant decrease in myelin thickness in Lkb1 -mutant animals (0.560±0.0072 in controls; 0.734±0.008 in mutants; mean±s.d., n =4 per group, P <0.0001). EM examination and G-ratio analysis also revealed that once myelinated, the axons of Lkb1 -mutant animals did not appear to lose myelin with age ( Fig. 2d–i ; G-ratio 0.631±0.0082 in P90 controls; 0.731±0.009 in P90 mutants; mean±s.d., n =4 per group, P <0.0001; and 0.650±0.007 in P150 controls; 0.740±0.0085 in P150 mutants; mean±s.d., n =3 per group, P <0.0001). 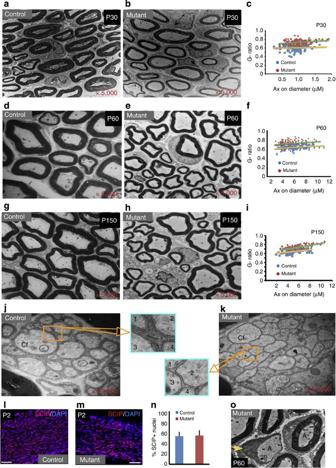Figure 2: Global PNS hypomyelination and C-fibre-sorting problems in theLkb1-mutant mice. Electron micrographs of cross-sections of 1-month-old (a,b), 2-month-old (d,e) and 5-month-old (g,h) control andLkb1-mutant sciatic nerves showing overall hypomyelination in theLkb1-mutant nerves. (c,f,i) Scatter plot displays G-ratios of individual axons as a function of the respective axon diameter. Over 100 axons from each of at least three control and three mutant animals per stage were analysed. (j,k) The structure of Remak bundle is abnormal inLkb1-mutant sciatic nerve. In Remak bundles, C-fibre axons (Cf) that are normally sorted by SC processes in control nerves (j) are unsorted and contact each other inLkb1-mutant nerves (k). Insets: higher magnification showing sorting of four axons (1–4) by control SC, but not byLkb1-mutant SC. (l) Representative images showing immunohistochemistry of longitudinal sections of postnatal day 2 control andLkb1-mutant sciatic nerves using SCIP (Oct6) antibody to mark SC nuclei and DAPI (to mark all nuclei) followed by fluorescence microscopy. (n) Quantitation of SCIP+nuclei showing no difference in the number of SCs between control andLkb1-mutant sciatic nerves (n=3 control and 3 mutant P2 nerves). (o) Electron micrograph of adultLkb1-mutant sciatic nerve showing survival of SCs. Asterisk showing an SC that myelinated an axon (A), while arrowhead shows an SC that survived but did not myelinate. Scale bar, 2 μM. Figure 2: Global PNS hypomyelination and C-fibre-sorting problems in the Lkb1 -mutant mice. Electron micrographs of cross-sections of 1-month-old ( a , b ), 2-month-old ( d , e ) and 5-month-old ( g , h ) control and Lkb1 -mutant sciatic nerves showing overall hypomyelination in the Lkb1 -mutant nerves. ( c , f , i ) Scatter plot displays G-ratios of individual axons as a function of the respective axon diameter. Over 100 axons from each of at least three control and three mutant animals per stage were analysed. ( j , k ) The structure of Remak bundle is abnormal in Lkb1 -mutant sciatic nerve. In Remak bundles, C-fibre axons (Cf) that are normally sorted by SC processes in control nerves ( j ) are unsorted and contact each other in Lkb1 -mutant nerves ( k ). Insets: higher magnification showing sorting of four axons (1–4) by control SC, but not by Lkb1 -mutant SC. ( l ) Representative images showing immunohistochemistry of longitudinal sections of postnatal day 2 control and Lkb1 -mutant sciatic nerves using SCIP (Oct6) antibody to mark SC nuclei and DAPI (to mark all nuclei) followed by fluorescence microscopy. ( n ) Quantitation of SCIP + nuclei showing no difference in the number of SCs between control and Lkb1 -mutant sciatic nerves ( n =3 control and 3 mutant P2 nerves). ( o ) Electron micrograph of adult Lkb1 -mutant sciatic nerve showing survival of SCs. Asterisk showing an SC that myelinated an axon (A), while arrowhead shows an SC that survived but did not myelinate. Scale bar, 2 μM. Full size image Small-caliber axons, usually <1 μM in diameter (called C-fibres), are normally associated with nonmyelinating SCs. These axons are normally bundled together by SCs to form Remak bundles. Within Remak bundles, SCs extend processes to sort individual C-fibres to prevent axon–axon contact. Ultrastructure analysis showed that Remak bundle axons in Lkb1 -mutant sciatic nerves contact each other, indicating that Lkb1 -mutant SCs fail to sort small axons ( Fig. 2j,k ). Interestingly, C-fibre-sorting problems have been recently reported in mice with SC-specific mitochondrial defects [2] , [3] , [25] . Hypomyelination was not due to reduced number of SCs in the premyelinating Lkb1 -mutant sciatic nerve; we found no differences in the number of SCIP + SCs between control and mutant animals ( Fig. 2l–n ). The percentage of proliferating SCs (as revealed by Ki67 immunohistochemistry) was also similar between genotypes ( Supplementary Fig. 3b–d ). Immunostaining with cleaved caspase-3 antibody did not show apoptosis of SCs in the Lkb1 -mutant sciatic nerve ( Supplementary Fig. 3e,f ). By EM, we could also detect individual SCs that failed to myelinate but survived in the adult Lkb1 -mutant sciatic nerve ( Fig. 2o ). Proliferation and survival of Lkb1 -mutant SCs was also normal in vitro confirming no significant cell-autonomous proliferation or survival defects ( Supplementary Fig. 3g,h ). Collectively, these results indicate that loss of SCs does not account for hypomyelination in Lkb1 -mutant mice. Impaired mitochondrial metabolism in Lkb1 -mutant peripheral nerves Appropriate myelination by SCs requires an accurately controlled genetic programme coordinated by a number of transcription factors including Egr2/Krox20, SOX10, SCIP/Oct6 and Nab1/Nab2 (refs 26 , 27 , 28 ). Egr2 controls several genes important for the formation of compact myelin. We therefore examined whether Lkb1 regulates the transcription of Egr2 or its target genes during myelination. Quantitative reverse transcriptase PCR (qRT–PCR) analysis showed that Egr2 and its transcripts including periaxin, myelin protein zero (MPZ) and myelin basic protein (MBP) increased during myelination; there were no significant differences between control and mutant nerves ( Fig. 3a ). Western blot analysis showed that myelin proteins were also present in normal amounts in the Lkb1 -mutant sciatic nerve ( Fig. 3b,c ), suggesting that the temporal regulation of myelin protein synthesis is not affected in Lkb1 -mutant PNS. 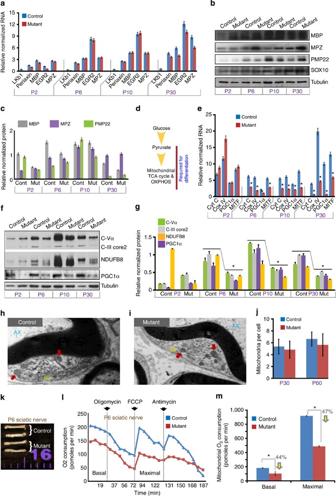Figure 3: Impaired mitochondrial metabolism inLkb1-mutant peripheral nerves. (a) qRT–PCR analysis of transcriptsLkb1and myelinating genes in the premyelinating (P2) and myelinating sciatic nerve. One pair of nerves from each of 3–6 animals was pooled to prepare RNA. (b) Western blots showing levels of myelinating proteins in the mouse sciatic nerve during myelination. (c) Quantitation of mean band intensities from two independent experiments shown. One pair of nerves from each of 6–10 animals was pooled. (d) Cartoon showing glucose metabolism. (e) qRT–PCR analysis showing transcripts of genes essential for mitochondrial oxidative metabolism in the mouse sciatic nerve (*P≤0.001). Error bars show s.d. Sciatic nerves from 3 to 6 mice per stage (two nerves per mice) were pooled and analysed in triplicate. (f) Western blot analysis showing that the levels of mitochondrial OXPHOS proteins increase during myelination in the mouse sciatic nerve. Protein lysates were made from pooled sciatic nerves of 6–10 mice per stage (two nerves per mice) for each experiment. (g) Quantitation of mean band intensities inffrom two independent experiments (*P≤0.001). (h,i) Representative electron micrographs showing SC mitochondria (red arrow) in control andLkb1-mutant sciatic nerves (Ax, axon). (j) EM sections (25–30) from 2 to 3 control or mutant mice were used. (k–m) Bioenergetic analysis of sciatic nerves: P6 sciatic nerves (k) were dissected and cut into equal lengths and subjected to bioenergetic analysis. Traces (l) and quantitation (m) of mitochondrial oxygen consumption of sciatic nerves. Error bars show s.d. (*P≤0.02). Data represent one out of four independent observations. During each experiment, 2–3 animals per genotype were used. Student’st-test was used to calculate statistical significance. Figure 3: Impaired mitochondrial metabolism in Lkb1 -mutant peripheral nerves. ( a ) qRT–PCR analysis of transcripts Lkb1 and myelinating genes in the premyelinating (P2) and myelinating sciatic nerve. One pair of nerves from each of 3–6 animals was pooled to prepare RNA. ( b ) Western blots showing levels of myelinating proteins in the mouse sciatic nerve during myelination. ( c ) Quantitation of mean band intensities from two independent experiments shown. One pair of nerves from each of 6–10 animals was pooled. ( d ) Cartoon showing glucose metabolism. ( e ) qRT–PCR analysis showing transcripts of genes essential for mitochondrial oxidative metabolism in the mouse sciatic nerve (* P ≤0.001). Error bars show s.d. Sciatic nerves from 3 to 6 mice per stage (two nerves per mice) were pooled and analysed in triplicate. ( f ) Western blot analysis showing that the levels of mitochondrial OXPHOS proteins increase during myelination in the mouse sciatic nerve. Protein lysates were made from pooled sciatic nerves of 6–10 mice per stage (two nerves per mice) for each experiment. ( g ) Quantitation of mean band intensities in f from two independent experiments (* P ≤0.001). ( h , i ) Representative electron micrographs showing SC mitochondria (red arrow) in control and Lkb1 -mutant sciatic nerves (Ax, axon). ( j ) EM sections (25–30) from 2 to 3 control or mutant mice were used. ( k – m ) Bioenergetic analysis of sciatic nerves: P6 sciatic nerves ( k ) were dissected and cut into equal lengths and subjected to bioenergetic analysis. Traces ( l ) and quantitation ( m ) of mitochondrial oxygen consumption of sciatic nerves. Error bars show s.d. (* P ≤0.02). Data represent one out of four independent observations. During each experiment, 2–3 animals per genotype were used. Student’s t -test was used to calculate statistical significance. Full size image A prerequisite to myelination is cell cycle exit and differentiation of SCs [27] . Recent studies in a number of cell types including ES cells and adipocyte, keratinocyte, neural and retinal ganglion precursor cells indicate that reprogramming of cellular metabolism is a required step for differentiation and tissue morphogenesis [8] , [9] , [10] , [11] , [12] . Proliferating cells are mainly glycolytic, and a transition from a glycolytic to mitochondrial oxidative metabolism {oxidative phosphorylation (OXPHOS)} occurs during differentiation ( Fig. 3d ). Proliferating SCs are also mainly glycolytic [29] . Although genes that regulate this metabolic transition are unknown, Lkb1 -null hematopoietic stem cells demonstrated reduced mitochondrial oxidative metabolism [17] . We therefore tested whether we could detect mitochondrial metabolism deficits in Lkb1 -mutant myelinating sciatic nerves. Remarkably, transcripts including mitochondrial transcription factors, co-activators and OXPHOS transcripts were all significantly downregulated in Lkb1 -mutant sciatic nerves ( Fig. 3e ). Western blot analysis confirmed that OXPHOS proteins were significantly upregulated during myelination in control sciatic nerves but considerably reduced in Lkb1 -mutant nerves ( Fig. 3f,g ). Because PGC1α, a master regulator of mitochondrial biogenesis, was reduced in Lkb1 -mutant sciatic nerve, we examined whether Lkb1 -mutant SCs have reduced number of mitochondria. However, mitochondrial count was not significantly different between adult control and mutant sciatic nerves ( Fig. 3h–j ). We therefore questioned whether mitochondria in Lkb1 -mutant sciatic nerves are functionally impaired. To determine this, we measured real-time oxygen consumption in P6 sciatic nerves ( Fig. 3k ) with the Seahorse XF analyzer. Remarkably, basal oxygen consumption was about 44% reduced, while uncoupled respiration (maximal mitochondrial oxygen consumption capacity) was about 47% reduced in Lkb1 -mutant nerves ( Fig. 3l,m ; four independent observations from four animals per genotype). These results suggest that, while mitochondrial metabolism is upregulated in the myelinating peripheral nerves (likely in the differentiating and myelinating SCs), this metabolic reprogramming is significantly impaired in the Lkb1 -mutant animals. Lkb1 regulates metabolic programming during SC differentiation Given the challenges of isolating the functional impairments to SC mitochondrial metabolism in vivo (because the nerves contain WT axons and mutant SCs), we conducted experiments in cultured SCs to unambiguously determine whether mitochondrial deficits are cell autonomous. We reasoned that if we could use an in vitro SC differentiation assay to define the metabolic shifts, we could determine whether SCs undergo metabolic transition during differentiation, and whether Lkb1 -mutant SCs are defective in this transition. Proliferating control and mutant SCs did not show any morphological differences ( Fig. 4a,c ). Alignment of Lkb1 -mutant SCs with axons (an indicator of SC–axon interaction) was also normal ( Supplementary Fig. 4a–d ). 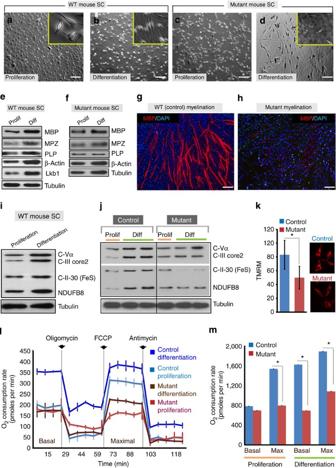Figure 4:Lkb1is required for optimal metabolic reprogramming during SC differentiation. (a–d) Bright-field images of proliferating and differentiating WT and mutant SCs. Inset shows spindle-shaped SCs with two or more short processes during proliferation, but with two long extended processes during differentiation. (e,f) Western bot analysis of SC proteins that increase duringin vitrodifferentiation. Tubulin was used as a protein loading control. Data are representative of three independent observations. (g,h) Representative images ofin vitromyelination in SC-DRG co-cultures established from control (g) andLkb1-mutant (h) mice. Myelination was confirmed by MBP immunofluorescence. Nuclei were stained by DAPI. Data are representative of three independent observations. (i,j) Western blot analysis showing that OXPHOS proteins are upregulated during differentiation of WT SCs but are largely blunted inLkb1-mutant SCs. Data are representative of three independent observations. (k) Trimethylrhodamine methyl ester fluorescence (inset) and quantitation shows mitochondrial membrane potential in control and Lkb1-mutant SCs (n=50–60 cells per genotype; error bars show s.d. (*P=0.02). Traces (l) and quantitation (m) demonstrating bioenergetic analysis of SCs during proliferation and differentiation: equal number of cells from each genotype was seeded in Seahorse XF analyzer 24-well plates and oxygen consumption was measured. Note: significant increase in basal and maximal oxygen consumption during differentiation of WT SCs, which is blunted inLkb1-mutant SCs. Also note that basal mitochondrial oxygen consumption of differentiating control SCs (dark blue line) reached close to their maximal capacity as carbonyl cyanide 4-(trifluoromethoxy) phenylhydrazone (FCCP) uncoupling only slightly increased oxygen consumption. This is unlike proliferating control SCs (light blue line) where basal oxygen consumption was about 50% of maximal. Data are representative of three independent observations; error bars show s.d. (*P≤0.001). Student’st-test was used to calculate statistical significance. Figure 4: Lkb1 is required for optimal metabolic reprogramming during SC differentiation. ( a – d ) Bright-field images of proliferating and differentiating WT and mutant SCs. Inset shows spindle-shaped SCs with two or more short processes during proliferation, but with two long extended processes during differentiation. ( e , f ) Western bot analysis of SC proteins that increase during in vitro differentiation. Tubulin was used as a protein loading control. Data are representative of three independent observations. ( g , h ) Representative images of in vitro myelination in SC-DRG co-cultures established from control ( g ) and Lkb1 -mutant ( h ) mice. Myelination was confirmed by MBP immunofluorescence. Nuclei were stained by DAPI. Data are representative of three independent observations. ( i , j ) Western blot analysis showing that OXPHOS proteins are upregulated during differentiation of WT SCs but are largely blunted in Lkb1 -mutant SCs. Data are representative of three independent observations. ( k ) Trimethylrhodamine methyl ester fluorescence (inset) and quantitation shows mitochondrial membrane potential in control and Lkb1-mutant SCs ( n =50–60 cells per genotype; error bars show s.d. (* P =0.02). Traces ( l ) and quantitation ( m ) demonstrating bioenergetic analysis of SCs during proliferation and differentiation: equal number of cells from each genotype was seeded in Seahorse XF analyzer 24-well plates and oxygen consumption was measured. Note: significant increase in basal and maximal oxygen consumption during differentiation of WT SCs, which is blunted in Lkb1 -mutant SCs. Also note that basal mitochondrial oxygen consumption of differentiating control SCs (dark blue line) reached close to their maximal capacity as carbonyl cyanide 4-(trifluoromethoxy) phenylhydrazone (FCCP) uncoupling only slightly increased oxygen consumption. This is unlike proliferating control SCs (light blue line) where basal oxygen consumption was about 50% of maximal. Data are representative of three independent observations; error bars show s.d. (* P ≤0.001). Student’s t -test was used to calculate statistical significance. Full size image Next, we verified the robustness of the in vitro differentiation system by examining three parameters: change in SC morphology (differentiating SCs extend actin polymerization-dependent long processes) [30] , upregulation of proteins associated with SC differentiation [31] , [32] , [33] , [34] and expression of SCIP/OCT6, a transcription factor important for myelinative differentiation [35] , [36] . Differentiating control and mutant SCs extended long processes ( Fig. 4a–d ), upregulated proteins that mark SC differentiation ( Fig. 4e,f ), and showed nuclear expression of SCIP/OCT6 ( Supplementary Fig. 4e–h ). Actin synthesis that is required for process extension was also noticed in differentiating SCs ( Fig. 4e ). Interestingly, Lkb1 protein expression was considerably increased during SC differentiation ( Fig. 4e ). In Lkb1 -mutant SCs, expression of differentiation markers increased, although that of proteolipid protein (PLP) did not ( Fig. 4f ). We next examined whether acute Lkb1 loss of function in WT SCs in vitro causes phenotypes similar to chronic loss of Lkb1 in SCs during development. Using lentiviral small hairpin RNA (shRNA), we silenced Lkb1 in WT mouse SCs ( Supplementary Fig. 4i ). Unlike Lkb1 -mutant SCs that proliferated similar to WT SCs, Lkb1 -silenced SCs showed a proliferative advantage over control {(nontarget (NT)} SCs ( Supplementary Fig. 4j ), indicating compensatory adaptive mechanisms during development in vivo . During in vitro differentiation, NT cells increased MBP and PLP expression ( Supplementary Fig. 4k ). Expression of these proteins remained unchanged in Lkb1- silenced cells. Given the hypomyelination of Lkb1 -mutant sciatic nerves, we wanted to examine whether the myelination defects persists in vitro independent of any potential systemic or central defects in Lkb1 -mutant animals. We co-cultured embryonic day 13.5 DRGs (that contains DRG neurons and SCs) from control and mutant mice and induced myelination by ascorbic acid. Immunocytochemistry with MBP antibody demonstrated that, while control SCs myelinated, Lkb1 -mutant SCs failed to myelinate DRG axons ( Fig. 4g,h ). Analogous to our in vivo observations, mitochondrial OXPHOS proteins increased during differentiation of WT SCs ( Fig. 4i ). As we predicted, Lkb1 -mutant SCs failed to upregulate OXPHOS proteins during differentiation ( Fig. 4j ). Impaired mitochondrial OXPHOS was also reflected by reduced mitochondrial membrane potential of Lkb1 -mutant SCs ( Fig. 4k ), a phenotype also reported in Lkb1 -null myeloid cells [17] . To examine whether these impairments have functional consequences, we conducted bioenergetic analysis of SCs during proliferation and differentiation by measuring oxygen consumption using the Seahorse XF analyzer ( Fig. 4l ; quantitation in Fig. 4m ). Basal oxygen consumption nearly doubled in control SCs during differentiation and this transition was blunted in Lkb1 -mutant SCs ( Fig. 4l,m ). Maximal respiration during proliferation and differentiation was also blunted in mutant SCs, suggesting reduced oxidative capacity of these cells. These results confirm that SCs undergo metabolic reprogramming during differentiation and that Lkb1 is required for this process. Collectively, our findings demonstrate that mitochondrial metabolism is required for myelination and that Lkb1 is crucial for optimal reprogramming of SC metabolism during differentiation and myelination. Reduced myelin lipid synthesis in Lkb1 -mutant sciatic nerves Proliferating cells including SCs are largely glycolytic. Thus, most of the glucose is incompletely oxidized to lactate through glycolysis. Less lactate is produced during differentiation as cells switch to mitochondrial metabolism and most of the glucose-derived pyruvate enters the TCA cycle ( Fig. 5a ). Because Lkb1 -mutant SCs demonstrated substantial defects in mitochondrial metabolism, we examined whether these cells are able to transit properly from glycolysis to mitochondrial metabolism during differentiation. Both WT and Lkb1 -mutant SCs showed high lactate to glucose ratio during proliferation ( Fig. 5b ) suggesting no difference in glycolysis. The lactate to glucose ratio decreased significantly in differentiating control SCs consistent with a reduction in glycolysis. Remarkably, Lkb1 -mutant SCs continued to produce increased amounts of lactate when induced to differentiate ( Fig. 5b ), indicating a failure to optimally transit to mitochondrial metabolism. As WT (control) SCs shifted to mitochondrial metabolism, they increased citrate production, which was blunted in Lkb1 -mutant SCs ( Fig. 5c ).These results were recapitulated when we silenced Lkb1 in WT SCs. During differentiation, while control (NT) SCs reduced lactate production ( Supplementary Fig. 4l ) and boosted citrate production ( Supplementary Fig. 4m ), these effects were blunted in Lkb1 -silenced SCs. NT cells upregulated OXPHOS proteins during differentiation ( Supplementary Fig. 4n ), which was significantly blunted in Lkb1 -silenced cells. These results confirm that unlike WT cells, SCs without Lkb1 do not adequately transit to mitochondrial metabolism during differentiation. 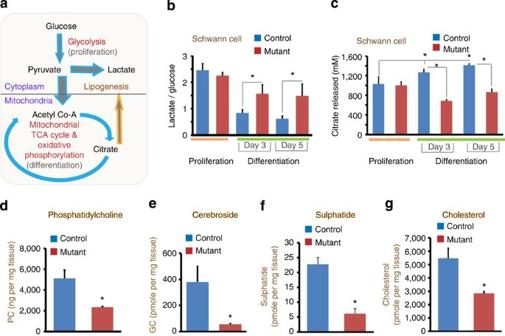Figure 5: Mitochondrial dysfunction leads to deficits in myelin lipid synthesis inLkb1-mutant sciatic nerves. (a) Cartoon showing metabolic shift of proliferating cells from glycolysis to mitochondrial metabolism during differentiation and its link tode novolipogenesis through production of citrate in the mitochondrial TCA cycle. (b) Lactate production by SCs as a function of glucose consumption during proliferation and differentiation. Equal number of cells was seeded in quadruplicate. Error bars show s.d. (*P≤0.003). Data represent three independent experiments. (c) Control SCs increased citrate production during differentiation, which was blunted inLkb1-mutant SCs. Data represent sextuplicate measurements from one of two independent experiments. Error bars show s.d. (*P≤0.0005). (d–g) Targeted mass spectrometry-based lipidomic analysis of P10 sciatic nerves done in a genotype-blinded manner. Error bars show s.d. (*P≤0.001). Data represent analysis of six pairs of control nerves (pooled) and three pairs of mutant nerves (pooled). Student’st-test was used to calculate statistical significance. Figure 5: Mitochondrial dysfunction leads to deficits in myelin lipid synthesis in Lkb1 -mutant sciatic nerves. ( a ) Cartoon showing metabolic shift of proliferating cells from glycolysis to mitochondrial metabolism during differentiation and its link to de novo lipogenesis through production of citrate in the mitochondrial TCA cycle. ( b ) Lactate production by SCs as a function of glucose consumption during proliferation and differentiation. Equal number of cells was seeded in quadruplicate. Error bars show s.d. (* P ≤0.003). Data represent three independent experiments. ( c ) Control SCs increased citrate production during differentiation, which was blunted in Lkb1 -mutant SCs. Data represent sextuplicate measurements from one of two independent experiments. Error bars show s.d. (* P ≤0.0005). ( d – g ) Targeted mass spectrometry-based lipidomic analysis of P10 sciatic nerves done in a genotype-blinded manner. Error bars show s.d. (* P ≤0.001). Data represent analysis of six pairs of control nerves (pooled) and three pairs of mutant nerves (pooled). Student’s t -test was used to calculate statistical significance. Full size image As cells transit to mitochondrial metabolism, pyruvate formed in glycolysis enters mitochondria to start the TCA cycle ( Fig. 5a ). Acetyl CoA formed from pyruvate condenses with mitochondrial oxaloacetate to form citrate. Citrate is further metabolized in the TCA cycle but is also exported to the cytosol where it is cleaved by ATP-citrate lyase (ACL) to form cytosolic acetyl CoA, the precursor for cellular lipids (fatty acids and cholesterol; Fig. 5a ). Deficiency in citrate production or ACL impairs de novo lipogenesis [37] , [38] . Because lipids account for 72–78% of the dry mass of PNS myelin [39] , and citrate production was impaired in Lkb1 -mutant differentiating SCs, we tested whether synthesis of myelin lipids is reduced in Lkb1 -mutant sciatic nerves. To examine this, we conducted targeted mass spectrometry-based lipidomic analysis of sciatic nerves at P10, when myelination is robust in mice. The main lipid classes in rodent PNS myelin are cholesterol (25–30%), phospholipids (~50% including 20% phosphatidylcholine (PC), 32–38% phosphatidylethanolamine and 10–35% sphingomyelin) and galactolipids (including 14–26% cerebrosides and 2–7% sulphalides) [39] , [40] . Most of these lipids are exclusively produced by SCs and deficiency in SC de novo lipogenesis causes severe peripheral neuropathy accompanied by hindlimb paralysis in humans and mice [39] , [41] . Analysis of mass spectrometry lipidomics data revealed that all the major myelin lipid classes were indeed greatly reduced in Lkb1 -mutant sciatic nerves ( Fig. 5d–g ; Supplementary Fig. 5a–d ). Consistent with existing literature [39] , phospholipids (which accumulate rapidly in the young sciatic nerve) and cerebrosides (which are low in the young nerve and accumulate gradually over 2 months) were found in similar proportions in the control P10 sciatic nerve (compare y axis in d versus e in Fig. 5 ). Our results are also in agreement with previous reports [39] showing that the large majority of peripheral nerve fatty acids in phospholipids are saturated and unsaturated long chains (16–18 carbon atoms; Supplementary Fig. 5a,b ), and that the most abundant fatty acid in cerebrosides are the very long-chain (20–24 carbon atoms) fatty acids ( Supplementary Fig. 5c ). Taken together, our results demonstrate that citrate-dependent lipid synthesis is significantly reduced during differentiation and myelination of Lkb1 -mutant SCs. Lkb1 regulates citrate synthase activity Citrate synthase (CS) is an evolutionarily conserved and pace-making enzyme of the TCA cycle. It regulates the critical and irreversible step of condensing one molecule of oxaloacetate with one molecule of acetyl CoA to form citrate. Because citrate production was consistently reduced in Lkb1 -mutant and -silenced cells, we sought to examine whether CS activity is comparable between Lkb1 -proficient and -deficient cells. We silenced Lkb1 in NIH 3T3 cells ( Fig. 6a , inset). Remarkably, Lkb1 silencing with three independent shRNA clones considerably reduced CS activity ( Fig. 6a ). 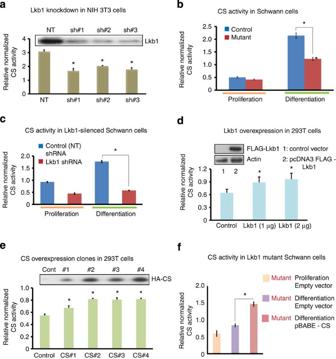Figure 6: Lkb1 regulates CS activity. (a) CS activity in NIH 3T3 cells stably infected with lentiviral NT shRNA or three independentLkb1shRNA clones. The extent of knockdown is shown by western analysis in inset (*P≤0.01). (b) CS activity duringin vitroproliferation and differentiation of WT (control) andLkb1-mutant SCs (*P=0.016). (c) CS activity duringin vitroproliferation and differentiation of WT SCs infected with NT orLkb1shRNA (*P=0.0004). (d) CS activity in HEK 293T cells transfected with empty vector or FLAG-tagged humanLkb1(*P≤0.002). (e) CS activity in HEK 293T cells transfected with four independent pBABE-puro CS clones (*P≤0.01). (f) CS activity inLkb1-mutant SCs infected with empty vector (control virus) or pBABE-puro-CS (*P=0.001). CS activities ina–fwere normalized to protein content of cell lysates and are expressed as nmol min−1per μg protein. Data are representative of two to three independent experiments. Error bars show s.d. Student’st-test was used to calculate statistical significance. Cont, control. Figure 6: Lkb1 regulates CS activity. ( a ) CS activity in NIH 3T3 cells stably infected with lentiviral NT shRNA or three independent Lkb1 shRNA clones. The extent of knockdown is shown by western analysis in inset (* P ≤0.01). ( b ) CS activity during in vitro proliferation and differentiation of WT (control) and Lkb1 -mutant SCs (* P =0.016). ( c ) CS activity during in vitro proliferation and differentiation of WT SCs infected with NT or Lkb1 shRNA (* P =0.0004). ( d ) CS activity in HEK 293T cells transfected with empty vector or FLAG-tagged human Lkb1 (* P ≤0.002). ( e ) CS activity in HEK 293T cells transfected with four independent pBABE-puro CS clones (* P ≤0.01). ( f ) CS activity in Lkb1 -mutant SCs infected with empty vector (control virus) or pBABE-puro-CS (* P =0.001). CS activities in a – f were normalized to protein content of cell lysates and are expressed as nmol min −1 per μg protein. Data are representative of two to three independent experiments. Error bars show s.d. Student’s t -test was used to calculate statistical significance. Cont, control. Full size image Consistent with a shift towards mitochondrial metabolism and citrate production, CS activity was significantly upregulated during differentiation of WT (control; Fig. 6b ) and NT shRNA (control) SCs ( Fig. 6c )—this effect was blunted in SCs with reduced or loss of Lkb1 . To determine whether there is a direct link between the levels of Lkb1 protein and CS activity, we overexpressed Lkb1 in HEK 293T cells (recall that Lkb1 protein levels increased during SC differentiation; Fig. 4e ). Expression of FLAG-tagged Lkb1 ( Fig. 6d , inset) increased CS activity in a dose-dependent manner ( Fig. 6d ). We argued that if reduced CS activity is an important cause behind differentiation defects of Lkb1 -mutant SCs, then normalizing CS activity or providing the CS substrate citrate in these cells could alleviate some of these defects. To explore this possibility, we cloned CS from NIH 3T3 cells. Four independent and sequence-verified HA-tagged retroviral CS clones were able to increase CS activity in 293T cells ( Fig. 6e and inset). Overexpressing one of these clones also increased CS activity in Lkb1 -mutant SCs ( Fig. 6f ) confirming enzymatic functionality of our CS clones. Restoring CS activity rescues defects of Lkb1 -mutant SCs Having confirmed the enzymatic activity of our CS clones, we sought to determine whether differentiation defects of Lkb1 -mutant SCs can be rescued by augmenting citrate levels. Our mass spectrometry results showed that lipids required for SC differentiation and myelination, including galactocerebrosides and sulphatides, are reduced in Lkb1 -mutant SCs. Therefore, we examined the expression of these two lipids in CS-expressing or citrate-fed Lkb1 -mutant cells during their differentiation. Proliferating mouse SCs in culture express very little of these lipids, but their expression is induced in high cyclic adenosine monophosphate (cAMP) conditions [42] (similar to our differentiating condition). Immunocytochemistry using antibodies against GalC (that detects galactocerebrosides) and O4 (that detects sulphatides) showed that WT SCs upregulate these lipids during differentiation in vitro ( Fig. 7a,b ; Supplementary Fig. 6a,b ). On the contrary, significantly fewer number of Lkb1 -mutant SCs could upregulate these lipids during differentiation ( Fig. 7c,d ; Supplementary Fig. 6c,d ). Remarkably, expressing CS in the mutant cells or adding the cell permeable citrate analogue methyl citrate to the culture media rescued expression of both lipids during differentiation ( Fig. 7e–g ; Supplementary Fig. 6e,f ). Restoring CS activity also normalized the levels of mitochondrial OXPHOS proteins in differentiating Lkb1 -mutant SCs ( Fig. 7h ). 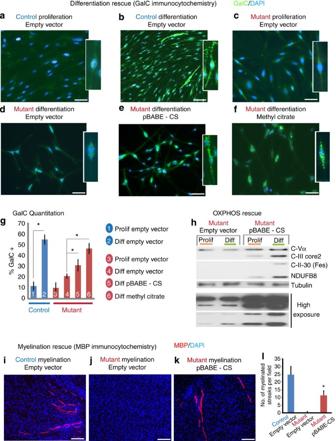Figure 7: Citrate restoration rescues differentiation and myelination defects ofLkb1-mutant SCs. (a–f) Immunocytochemistry with GalC antibody in proliferating (Prolif) and differentiating (Diff) control orLkb1-mutant SCs.Lkb1-mutant SCs were infected with control retrovirus (empty vector) or pBABE-CS or fed with methyl citrate. Nuclei were stained with 4',6-diamidino-2-phenylindole (DAPI). (g) Quantitation of GalC-positive SCs in experiments (a–f). Error bars show s.d. (*P≤0.02). Data are representative of two independent experiments—for each experiment, quadruplicates for each condition was used. (h) Western blot analysis showing levels of OXPHOS proteins in proliferating and differentiatingLkb1-mutant SCs that were infected with control virus (empty vector) or pBABE-CS retrovirus. A high exposure of the OXPHOS blots shows that OXPHOS proteins are expressed inLkb1-mutant (empty vector) cells, but in very low amounts and that the majority of them are not upregulated during differentiation. (i–k) MBP immunocytochemistry showingin vitromyelination and its quantitation (l; *P=0.02) in SC-DRG co-cultures from control andLkb1-mutant mice. Control SCs were infected with control retrovirus (empty vector) in co-cultures. Mutant SCs were infected with control virus or pBABE-CS. Nuclei were stained with DAPI. Data are representative of two independent experiments containing five control and three mutant animals; quadruplicates for each condition were examined from each experiment. Student’st-test was used to calculate statistical significance. Scale bar, 02 μM (a–f); 2 μM (i–k). Figure 7: Citrate restoration rescues differentiation and myelination defects of Lkb1 -mutant SCs. ( a – f ) Immunocytochemistry with GalC antibody in proliferating (Prolif) and differentiating (Diff) control or Lkb1 -mutant SCs. Lkb1 -mutant SCs were infected with control retrovirus (empty vector) or pBABE-CS or fed with methyl citrate. Nuclei were stained with 4',6-diamidino-2-phenylindole (DAPI). ( g ) Quantitation of GalC-positive SCs in experiments ( a – f ). Error bars show s.d. (* P ≤0.02). Data are representative of two independent experiments—for each experiment, quadruplicates for each condition was used. ( h ) Western blot analysis showing levels of OXPHOS proteins in proliferating and differentiating Lkb1 -mutant SCs that were infected with control virus (empty vector) or pBABE-CS retrovirus. A high exposure of the OXPHOS blots shows that OXPHOS proteins are expressed in Lkb1 -mutant (empty vector) cells, but in very low amounts and that the majority of them are not upregulated during differentiation. ( i – k ) MBP immunocytochemistry showing in vitro myelination and its quantitation ( l ; * P =0.02) in SC-DRG co-cultures from control and Lkb1 -mutant mice. Control SCs were infected with control retrovirus (empty vector) in co-cultures. Mutant SCs were infected with control virus or pBABE-CS. Nuclei were stained with DAPI. Data are representative of two independent experiments containing five control and three mutant animals; quadruplicates for each condition were examined from each experiment. Student’s t -test was used to calculate statistical significance. Scale bar, 02 μM ( a – f ); 2 μM ( i – k ). Full size image We next examined whether CS expression or methyl citrate feeding rescues myelination defects of Lkb1 -mutant SCs. In DRG axon co-cultures from control mice, SCs differentiated and myelinated axons as revealed by the expression of MBP ( Fig. 7i ) and GalC ( Supplementary Fig. 7a ). These markers were virtually absent in co-cultures from Lkb1 -mutant mice infected with empty vector ( Fig. 7j ; Supplementary Fig. 7b ). In Lkb1 -mutant co-cultures in which proliferating SCs were infected with pBABE-puro-CS retrovirus before induction of myelination ( Fig. 7k,l ; Supplementary Fig. 7c ), expression of MBP and GalC was partially restored. Although methyl citrate was tolerated by SCs during their differentiation (3 days), DRG axons deteriorated during the 2-week myelination assays and myelination per se was blocked in all cultures. Collectively, our data show that a deficit in Lkb1 -regulated metabolic reprogramming during SC myelination results in inadequate myelin lipid synthesis leading to hypomyelination and peripheral neuropathy of Lkb1 -mutant mice ( Fig. 8 ). This metabolic reprogramming is likely regulated by many genes, important among which is the tumour suppressor Lkb1 . We found that by regulating CS activity, Lkb1 mediates the metabolic shift during SC differentiation and myelination. 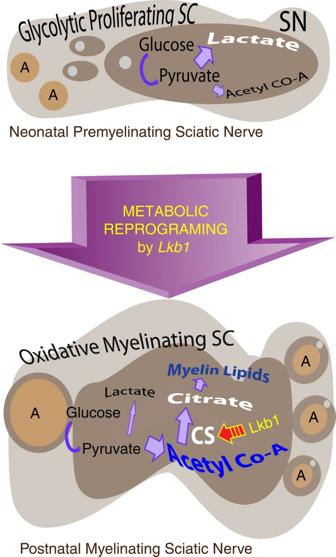Figure 8: Schematic showing the role ofLkb1in PNS myelination. In the premyelinating sciatic nerve (SN, light brown), axons (A) are unmyelinated and SC (brown oval) proliferate and meet their bioenergetic demands largely through glycolysis, producing more lactate compared with the mitochondrial TCA cycle metabolite acetyl CoA.Lkb1augments CS activity to reprogram metabolism from glycolytic to oxidative (mitochondrial) allowing SCs to differentiate and start myelinating axons (A). During this metabolic shift, glucose is fully oxidized through the TCA cycle and OXPHOS producing more acetyl CoA than lactate. Acetyl CoA condenses with oxaloacetate (not shown) to form citrate, which is exported to the cytoplasm to initiatede novosynthesis of myelin lipids. Figure 8: Schematic showing the role of Lkb1 in PNS myelination. In the premyelinating sciatic nerve (SN, light brown), axons (A) are unmyelinated and SC (brown oval) proliferate and meet their bioenergetic demands largely through glycolysis, producing more lactate compared with the mitochondrial TCA cycle metabolite acetyl CoA. Lkb1 augments CS activity to reprogram metabolism from glycolytic to oxidative (mitochondrial) allowing SCs to differentiate and start myelinating axons (A). During this metabolic shift, glucose is fully oxidized through the TCA cycle and OXPHOS producing more acetyl CoA than lactate. Acetyl CoA condenses with oxaloacetate (not shown) to form citrate, which is exported to the cytoplasm to initiate de novo synthesis of myelin lipids. Full size image In this study, we examined the function of the metabolic kinase Lkb1 in SC differentiation and myelination by ablating its function in myelinating glia. We show that proliferating SCs are primarily glycolytic and differentiating SCs shift to a mitochondrial oxidative metabolism by increasing CS activity, flux through TCA cycle and augmenting mitochondrial oxygen consumption. We found that Lkb1 -null SCs cannot fully augment CS activity and are unable to fully transit from glycolytic to oxidative metabolism during differentiation. Reduced CS activity resulted in inadequate production of citrate, decreased flux through the TCA cycle and reduced mitochondrial oxygen consumption and membrane potential. Inadequate production of citrate, a precursor for de novo lipogenesis, had profound effects on myelination as synthesis of myelin lipids was greatly reduced leading to hypomyelination in Lkb1 -mutant PNS. The extent of hypomyelination was sufficient to reduce CMAP during electrical stimulation of the sciatic nerve, which leads to muscle atrophy, hindlimb weakness, diminished locomotion, peripheral neuropathy and premature death of Lkb1 -mutant mice. The importance of axonal mitochondria in peripheral neuropathies is known [1] . The contribution of SC mitochondria for myelin formation and maintenance, and how this function is crucial to preserving axonal integrity is only recently being elucidated. In these recent studies, SC-specific loss of the mitochondrial transcription factor A gene ( Tfam ) [2] , [3] or SC/oligodendrocyte-specific loss of Cox10 , a gene necessary for assembly of mitochondrial cytochrome oxidase [25] , caused PNS hypomyelination and peripheral neuropathy. However, little is known how SC mitochondrial functions are integrated with SC proliferation, differentiation and PNS myelination during development. For example, while it is known that during the early neonatal period proliferating mouse SCs exit cell cycle, synthesize basement membrane and begin to myelinate peripheral axons [43] , the cell-intrinsic mechanisms regulating the transition of SCs from a proliferative to a non-proliferative, myelinating state are not well understood. One recently appreciated mechanism is that a change in cellular bioenergetics occurs during cellular differentiation and this change is a required event for differentiation [9] , [10] , [11] , [12] . However, whether SCs undergo such bioenergetic shift is unknown. Moreover, our knowledge about the genes that regulate this transition is limited. We show here that Lkb1 is a gene that regulates the bioenergetic shift during SC differentiation and myelination. Besides its tumour suppressor properties, Lkb1 performs many other functions important for the normal biology of cells. We show that Lkb1 loss affects the bioenergetics of SCs. The bioenergetics of proliferating Lkb1 -mutant SCs at the basal level did not change as revealed by similar lactate production (a measure of glycolysis) and mitochondrial oxygen consumption. This glycolytic metabolism of proliferating SCs, as reported by others [29] , [44] , presumably allowed the generation of normal number of SCs in the premyelinating sciatic nerve of Lkb1 -mutant mice. However, basal respiration during differentiation [45] , [46] , [47] , which increased nearly twofold in control SCs, as well as mitochondrial respiratory capacity were severely diminished in both proliferating and differentiating Lkb1 -mutant SCs. This diminished mitochondrial oxidative metabolism lead to improper SC differentiation and hypomyelination in the Lkb1 -mutant animals. It is interesting that, while myelin lipids were greatly reduced, myelin proteins were present in near normal amounts in the Lkb1 -mutant sciatic nerve. Thus, Lkb1 loss in SCs does not significantly affect transcription, translation or stability of myelin proteins in vivo . Mice with myelinating glia-specific disruption of cholesterol synthesis (squalene synthase knockout) have thinner myelin, although its ultrastructure, lipid and protein composition were not affected. This suggests that protein levels are likely regulated based on available myelin lipids [45] . It remains to be examined whether Lkb1 mutants have ultrastructural abnormalities in PNS myelin, since cholesterol regulates intracellular trafficking of myelin proteins [46] . Lipids constitute 70–80% of myelin. The extraordinarily high level of lipid synthesis required for myelination makes this process highly vulnerable to defects in lipid metabolism as observed in numerous inherited lipid disorders in humans that cause myelin abnormalities and peripheral neuropathy (for example, Krabbe disease, Tangier disease, metachromatic leukodystrophy, Refsum disease) [47] . Given the central role of lipids in normal SC biology, in determining myelin thickness and in human-inherited myelination disorders, and because mice with mitochondrial defects demonstrated aberrant SC lipid metabolism [3] , and because Lkb1 mutant SCs produced insufficient amounts of citrate, the precursor to de novo lipogenesis, we interrogated whether myelin lipids were present in normal amounts in Lkb1 -mutant sciatic nerves. The remarkable reduction of the major lipid classes in the Lkb1 -mutant sciatic nerve suggests that the defect is likely upstream of citrate production because de novo fatty acid synthesis initiates from citrate. Therefore, restoring CS expression in Lkb1 -mutant SCs normalized myelin lipid production. We cannot rule out at this time that CS is an indirect target of Lkb1 or restoring CS activity improves general mitochondrial function and Lkb1 has other targets upstream of CS. Further studies are necessary to address these questions. We chose GalC and O4 to detect galactocerebrosides and sulphatides—two lipids predominantly expressed during myelin-related differentiation of glial cells [48] , [49] . GalC is not detected in cultured proliferating mouse SCs and is induced specifically under non-proliferating myelin-related differentiating conditions [49] . O4 expression is on the otherhand unstable (high in late embryonic nerves, decreases during in vitro culture and re-induced by cAMP) [42] . O4 is an early SC differentiation marker in vivo [49] and cAMP (present in our differentiating medium) triggers differentiation of SCs to O4-positive early differentiation stage [49] . Our in vitro analysis using these two markers suggests that Lkb1 likely regulates the initial transition of SCs from proliferation to an early differentiation stage, although we cannot exclude that it also regulates later steps of SC myelin-related differentiation. Myelination was however not completely normalized in CS-overexpressing Lkb1-mutant co-cultures and this could be due to various reasons. First, co-cultures had to be infected with a virus that infects only proliferating cells (retrovirus and SCs in this case) to circumvent infection of DRG neurons, and retroviral infection of DRG-SC co-cultures itself reduced overall myelination. Second, infected SCs could not be selected with puromycin, which would otherwise kill DRG neurons. This precluded us from determining the efficiency of retroviral infection. In conclusion, we demonstrate that Lkb1 controls cellular lipid levels by positively regulating CS activity. Recent reports show that lipogenesis was also reduced in Lkb1 -knockout white adipose tissue [19] and Lkb1 -knockout muscle displayed reduced CS activity [50] . That the defect in Lkb1 -mutant SCs is likely at the level of CS is corroborated by the reversal of lipid levels by methyl citrate during in vitro differentiation and myelination. Further studies will be needed to examine whether Lkb1 regulates PNS myelination by regulating CS activity directly or through one of its 14 downstream kinase substrates. In summary, our study shows that Lkb1 , a widely known tumour suppressor gene, plays an unexpected and important role in SC differentiation and myelination through regulation of mitochondrial metabolism and de novo lipogenesis. Regulation of mitochondrial OXPHOS and de novo lipogenesis by Lkb1 may have broader implications not only in normal development but also in metabolic reprogramming in human pathologies including functional regeneration of axons after injury and in demyelinating neuropathies. Generation of Lkb1 -conditional knockout mice All animal procedures were carried out in accordance with the Institutional Animal Care and Use Committee-approved protocol of Cincinnati Children’s Hospital and Medical Center. Animals were maintained in 12 h light/dark cycle and monitored daily by an animal care personnel. Animals were raised in a mixed C57BL/6 and fetal bovine serum (FVB) background. Animals were maintained up to four animals per cage. Both males and females were used as control or experimental animals. Animals for this study were generated by breeding Lkb1 lox/− or LKB1 lox/lox females provided by Ronald A. Depinho (MD Anderson Cancer Center, Houston, TX) with Cnp-Cre + male mice obtained from Klaus-Armin Nave (Max Planck Institute of Experimental Medicine, Gottingen, Germany). The Lkb1 -null allele was generated in the DePinho laboratory by crossing Lkb1 lox mice with EIIa-Cre mice. Experimental mice were Lkb1 lox/lox ; Cnp-Cre + or LKB1 lox/− ; Cnp-Cre + and control mice were LKB1 lox/+ ; Cnp-Cre + , LKB1 lox/lox ; Cnp-Cre − or LKB1 lox/− ; Cnp-Cre − . The following primers were used for genotyping: Lkb1 null forward: 5′-GGGCTTCCACCTGGTGCCAGCCTGT-3′, Lkb1 WT forward: 5′-GATGGAGGACCTCTTGGCCGGCTCA-3′, Lkb1 (common reverse for null and WT, and forward for lox ): 5′-GAGATGGGTACCAGGAGTTGGGGCT-3′, Lkb1 lox reverse: 5′-TCTAACAATGCGCTCATCGTCATCCTCGGC-3′, Cre forward: 5′-ATGAGTGAACGA ACCTGGTCGAAA-3′ and Cre reverse: 5′-GCAGAACCTGAAGATGTTCGCGAT-3′. Sciatic nerve dissection Sciatic nerves were grasped with a pair of forceps and cut from the spine to the knee with a pair of spring scissors. All dissected tissues were either used fresh or saved at −80 °C until use. Nerve histology Nerves from control and Lkb1 -mutant animals were embedded in 100% epoxy. Thick sections (1 mm) were prepared for toluidine blue staining and light microscopy. Electron microscopy Mice were anaesthetized and perfused with EM fixative (4% paraformaldehyde, 2.5% glutaraldehyde, phosphate-buffered saline, pH 7.4–7.6). Tissues were post-fixed in EM fixative buffer before washing in 0.1 M Na cacodylate buffer (EMS, Hatfield, PA) and post-fixed in 1% osmium tetroxide (OsO 4 , EMS) for 1 h at 4 °C. Samples were washed again in 0.1 M Na cacodylate buffer followed by dehydration through graded series of ethanol. Samples then were embedded in LX-112 (Ladd Research Industries, Williston, VT). Sciatic nerves were cut with an ultramicrotome (Leica EM UC7, Buffalo Grove, IL) at 90 nm thickness. Sections were counterstained with uranyl acetate 2% (EMS) and lead citrate. All images were taken using a 120-kV transmission electron microscope (Hitachi, H-7650, V01.07, Tokyo, Japan). Extracellular recordings Dissection of spinal cords and recoding were done as described [51] , [52] . Briefly, after perfusion, spinal cords from P6 newborn pups were removed and hemisectioned in artificial cerebrospinal fluid (aCSF) containing: NaCl (127 mM), KCl (1.9 mM), KH 2 PO 4 (1.2 mM), CaCl 2 (2 mM), MgSO 4 (1 mM), NaHCO 3 (26 mM) and D -glucose (20.5 mM) with oxygenated air (95%O 2 /5%CO 2 ). After dissection, spinal cords were moved to aCSF-containing bath. Using tightly fitting glass pipets, dorsal roots were stimulated (0.3–0.6 mA, S88X, SIU-C, Grass technologies). Extracellular potentials are recorded from ventral roots (L4 and L5) using tightly fitting glass pipets with pre-amplifier (P55, Astro-Med) and digitizer (Digidata 1440A, Molecular Devices) and a data acquisition programme (Clampex version 10, Molecular Devices). Recorded traces are averages of 20 individual stimuli applied at 0.1 Hz. CMAP recording To analyse nerve conduction and muscle function, single CMAPs were recorded in vivo from the lateral gastrocnemius muscles of anaesthetized mice during electrical stimulation of the sciatic nerve. Control and Lkb1 -mutant mice were anaesthetized with an intraperitoneal injection of 50 mg kg −1 sodium phenobarbital. Then, the lateral gastrocnemius muscle was exposed from the knee to ~4 mm above the ankle. Next, the sciatic nerve was exposed near the biceps femoris muscles. Mylar-coated steel recording wires (California Fine Wire) were implanted into the lateral gastrocnemius muscles and ground wires were inserted under the skin near the ankle. A concentric bipolar stimulating electrode was placed on the sciatic nerve and used for electrical activation. CMAPs were amplified and obtained using a Micro 1401 data acquisition unit and analysed using Spike 2 software (Cambridge Electronic Design, Cambridge, UK). A 2–4 mA electrical stimulation of the sciatic nerve immediately proximal to the tibial, sural and common peroneal branches was employed via a stimulus isolation unit (WPI) connected to the Micro 1401. In addition to isolated electrical stimulation, a 10-s train of pulses were delivered to the sciatic nerve at 1 Hz (0.2 ms duration) at the described current intensities. After recording, the sciatic nerve was axotomized and stimulation of the proximal end of the sciatic nerve was performed to ensure CMAPs were generated from direct nerve stimulation. CMAP amplitude and duration were calculated from each stimulation paradigm. The average of the stimulations of the sciatic nerve for each paradigm was obtained and then averaged across animals. RNA preparation and qRT–PCR RNA was extracted by adding 350 μl RLT buffer to each sample using Qiagen RNeasy mini kit (Qiagen, Valencia, CA) according to manufacturer’s instructions. Complementary DNA was made with ABI high Capacity cDNA Kit (ABI, Life Technologies, Grand Island, NY) and stored at −80 °C. qRT–PCR analysis was performed using SYBR green methodology using ABI SYBR green PCR master mix (ABI, Life Technologies) in a 7500 real-time PCR machine (Applied Biosystems, Grand Island, NY, 7500 Real-Time PCR System V1.4.0). Results were expressed as relative normalized RNA (expressed in arbitrary units) by calculating the ratios of crossing points of amplification curves of target genes’ cDNA and internal standard using the RelQuant software (Roche Diagnostics). The following primers were used: MBP: 5′-CCCTGGCCATTGTGGTTTAC-3′ and 5′-CCATTCACTGGACCAGAAGGAG-3′; MPZ: 5′-GACCCTGCACTGCTCCTT-3′ and 5′-GTCCCTTGGCATAGTGGAA-3′; periaxin: 5′-GGCAGCTAAGAGCCTCAGCTT-3′ and 5′-CTTGTAGGGCTCTGCGCATT-3′; EGR2: 5′-CTGGGAGGCCCCTTTGAT-3′ and 5′-GGAGATCCAAGGGCCTCTTC-3′; cytochrome C: 5′-GGAGGCAAGCATAAGACTGG-3′ and 5′-TCCATCAGGGTATCCTCTCC-3′; cytochrome C oxidase IV (Cox4): 5′-AGAAGGAAATGGCTGCAGAA-3′ and 5′-GCTCGGCTTCCAGTATTGAG-3′; β-actin: 5′-GACATGGAGAAGATCTGGCA-3′ and 5′-GGTCTCAAACATGATCTGGGT-3′; Lkb1: 5′-AAGGCTGTTTGTGTGAATGGC-3′ and 5′-TCCTGATGACACACTGTAGGCC-3′; and PGC1α: 5′-ACTATGAATCAAGCCACTACAGAC-3′ and 5′-TTCATCCCTCTTGAGCCTTTCG-3′. Western blot analysis Cells or sciatic nerves were lysed in RIPA buffer and western blot analysis was done as described [53] . Briefly, cells or sciatic nerves were triturated in RIPA buffer, following centrifugation at 14,000 r.p.m. for 10 min at 4 °C. Protein content of lysates was determined by the bicinchoninic acid (BCA) protein assay kit (PI23235, Thermo Science, Waltham, MA) and resolved on SDS–polyacrylamide gel electrophoresis gel. After blocking in 5% dry milk in Tris-buffered saline, blots were incubated overnight at 4 °C with primary antibodies, washed three times with Tris-buffered saline with Tween 20and incubated with horseradish peroxidase -linked secondary antibodies (Cell Signaling Technology, Danvers, MA). Detection was done by the horseradish peroxidase chemiluminescent reagent (WBKLS0100, Millipore, Darmstadt, Germany). The following antibodies were used: beta actin (#4790; dilution 1:2,000), LKB1 (#3047; dilution 1:1,000), alpha tubulin (#3873; dilution 1:2,000; all from Cell Signaling Technology), MBP (SMI99; dilution 1:1,000; Covance, Princeton, NJ), P0 (PZO0308; dilution 1:500) and PLP (PLP; dilution 1:1,000; Aves Labs, Tigard, OR), OXPHOS antibody cocktail (458099; dilution 1:2,000; Life Technologies), PGC1alpha (#AB54481; dilution 1:1,000, Abcam, Cambridge, MA), SOX10 (sc-17342; dilution 1:500; Santa Cruz Biotechnology, Santa Cruz, CA) and PMP22 (P0081; dilution 1:1,000; Sigma, St Louis, MO). Most antibodies were validated by using multiple positive and negative control tissues. Lkb1 antibody was validated by using Lkb1-proficient and -deficient lung cancer cells. Original X-ray films of western blots are shown in Supplementary Fig. 8 . Immunofluorescence microscopy Tissue processing for frozen sections was done as before [53] . Briefly, mice were perfused transcardially with phosphate-buffered saline (PBS) and 4% paraformaldehyde (PFA) in PBS. After overnight post fixation in 4% PFA at 4 °C, tissues were transferred into 20% sucrose for at least 36 h before embedding into optimum cutting temperature (OCT) medium. Cryostat sections (12 μm) of sciatic nerves were dried at room temperature (RT) for 15 min, fixed in 4% PFA for 15 min at RT and permeabilized with 0.25% Triton X-100 in PBS. Blocking was done with 10% horse serum followed by incubation with primary antibody overnight at 4 °C. Cultured SCs were processed similarly. The following antibodies were used: LKB1 clone 5c10 (05–832; dilution 1:100; from Upstate Biotechnology, now EMD Millipore, Billerica, MA), α-tubulin (3873; dilution 1:2,000), cleaved caspase-3 (9661; dilution 1:1,000; Cell Signaling Technology), Cre (69050; dilution 1:1,000; Novagen, now EMD Millipore, Billerica, MA), MBP (SMI99; dilution 1:1,000; Covance), SCIP (sc-11661; dilution 1:200; Santa Cruz Biotechnology and also a gift from John Bermingham), Ki76 (VP-K452; dilution 1:500; Vector Laboratories, Burlingame, CA), neurofilament (2837; Sigma), NeuN (MAB377; dilution 1:1,000; Chemicon, now Millipore), S100β (ZO311; dilution 1:1,000; Dako, Carpinteria, CA), O4, clone 81 (MAB345) and Gal-C (MAB342; dilution 1:500; EMD Millipore, St Louis, MO). All fluorescent images were captured with Leica microscope (Leica DMI6000) using Openlab (Improvision V5.5.0) software. Cell culture DRG and SC culture . DRG and SC cultures were obtained from E12.5 or E13.5 embryonic spinal cords dissected in L15 medium on ice [54] . DRGs were seeded into poly- L -lysine (PLL; R&D, Minneapolis, MN) and laminin (Life Technologies)-pre-coated 24-well plate in neurobasal media containing 50X B27 (Life Technologies), 200 μg ml −1 nerve growth factor (NGF) (Harlan, Indianapolis, IN), 10% horse serum (Life Technologies), 2 mM glutamine (Life Technologies) and penicillin/streptomycin (Thermo Scientific). The culture was checked daily and half of the media were changed every 2 days. Cultures were maintained either as neuron-SC co-cultures (for in situ myelination experiments) or were processed to obtain pure DRG or SC cultures. After 2 weeks, DRG explants (containing DRG neurons) from 7 to 10 days old co-cultures were cut right at the periphery where axons sprout from the DRG neurons and removed. These DRG neurons were used for western blot analysis. SCs growing along with the axonal mesh were lifted and dissociated in 1 mg ml −1 collagenase and 0.05% trypsin with EDTA for 30 min at 37 °C, neutralized with serum-containing media and triturated 30 times. SCs were seeded into the PLL-coated plates in DMEM media (Thermo Scientific) with 10% primary serum (Gemcell US origin fetal bovine serum, Gemini, West Sacramento, CA), 2 mM L -glutamine (Life Technologies) and 1% penicillin/streptomycin. The following day, culture medium was replaced with medium containing 100 μM cytosine arabinoside (Sigma) to prevent proliferation of non-neuronal cells. Most of the contaminating fibroblasts were eliminated by incubating cells during passaging with Thy1.2 antibody (Mouse CD90.2 antibody, Becton Dickenson, Heidelberg, Germany). After 3 days, pure SCs were washed and replaced with DMEM containing 10% primary serum and 2 mM L -glutamine with adding 10 ng ml −1 HRG1-β1 epidermal growth factor (EGF) domain (R&D) and 2.5 μM forskolin (Sigma) and 100 mM bovine pituitary extract (Life Technologies) to allow SC proliferation. For SC differentiation, proliferation media were changed to DMEM without serum for 12 h and 1 mM dibutyryladenosine 3′:5′ cAMP (Sigma) was added for cells to differentiate for 3–5 days. In some of LKB1 -mutant wells, trisodium (2RS,3RS)-2-methylcitrate (Sigma) was added after removing glutamine from culture media [55] . NIH 3T3 and HEK293 cells were gown in DMEM media (Thermo Scientific) with 10% fetal bovine serum (Life Technologies). CS cloning . Total RNA was extracted from NIH 3T3 cells using Qiagen RNeasy Mini Kit (Qiagen) according to manufacturer’s instructions. cDNA was made using ABI High Capacity cDNA Kit (ABI, Life Technologies). Restriction sites and a C-terminal HA tag were added by PCR using the following primers: forward 5′-GTACGAATTCATGGCTCTACTCACTGCAGC-3′ and reverse 5′-GAAGTTTGTGGACTCTAAGTACCCATACGA TGTTCCAGATTACGCTTAAGTCGACGTAC-3′. The PCR product and the recipient plasmid pBABE-puro empty backbone (Addgene, Cambridge, MA) were digested with EcoRI and SalI. The ligation reaction was transformed into GC10 Competent Cells (Sigma), and plasmid DNA was purified with QIAGEN Hi Speed Plasmid Midi Kit (Qiagen). 293T cells were used for DNA transfection with pBABE-puro-CS or pBABE-puro empty vector using Polyplus jetPRIME (Polyplus Transfection, New York, NY). Transfection . 293T cells were transfected with pcDNA3-FLAG-Lkb1 or control (empty vector) plasmids (gift from Reuben Shaw, Salk Institute) to overexpress Lkb1. pBABE-puro-CS or empty vector plasmids were used to overexpress CS. Transfection was done using Polyplus jetPRIME (Polyplus Transfection). LKB1 knockdown and lentivirus preparation . The following LKB1 shRNA clones were purchased from the Lenti shRNA Library Core (Cincinnati Children’s Hospital Medical Center (originally from the Sigma Mission RNAi validated genome-wide The RNAi Consortium shRNA library)): clone1 (TRCN0000024144), clone2 (TRCN0000024145), clone3 (TRCN0000024146), clone4 (TRCN0000024147), clone5 (TRCN0000024145) and the sequences that exhibited maximal knockdown were used for the study. Plasmids were made using Sigma GenElute HP Plasmid midiprep kit (Sigma) and Lkb1 shRNA or control (NT shRNA) viruses were made in 293T cells using Polyplus jetPRIME (Polyplus Transfection) following manufacturer’s instructions. Infected cells were selected by adding puromycin 3 days after infection and knockdown efficiency was examined by western blot using Lkb1 antibody. Lentivirus infection of SCs . For CS overexpression in SCs, pBABE-puro-CS retrovirus was made as above. SC-DRG co-cultures or purified SCs were infected twice with either pBABE-puro empty vector or pBABE-puro-CS-concentrated virus during SC proliferation. Purified SCs were selected with puromycin (1 mg ml −1 ) before differentiation experiments. In vitro myelination . Myelination was initiated in 2-week-old co-cultures as described by Päiväläinen et al. [56] , by adding 5% horse serum, 50 μg ml −1 ascorbic acid (Sigma) and 0.5 μM forskolin. Half of the media were changed every third day. Myelination was continued for 2 weeks. In vitro cell proliferation and survival . Cell proliferation was measured with CellTiter-Fluor Assay kit (Promega, Madison, WI). Briefly, equal numbers of cells were seeded in triplicate and readings were taken on 24, 48 and 72 h after seeding. Cell survival was measured by trypan blue exclusion method. Oxygen consumption rate of sciatic nerves Sciatic nerves were dissected from P6 animals on ice, aligned next to a ruler, trimmed to equal lengths (about 3 mm) and immediately transferred into the seahorse assay medium (aCSF with 0.4% bovine serum albumin+10 mM glucose+0.25 mM pyruvate) [57] , [58] in 10 cm petri dish. To immobilize nerves, 10 μl of chicken plasma (Cocalico Biologicals, Reamstown, PA) was added on a nylon capture screen (Seahorse Biosciences, North Billerica, MA) and the nerve was layered in the centre of the screen and stretched well. Thrombin (5 μl) from bovine plasma (Sigma) was added to initiate clotting and immobilize nerves. After 2 min, the screens with the tissue were put upside down into the XF24 islet capture plate containing assay medium. Slices in XF Islet Capture Microplates were incubated in a CO 2 -free incubator at 37 °C for 1 h to allow temperature and pH equilibration and then loaded into a XF24 machine (Seahorse Bioscience) to measure oxygen consumption rate. Drugs (oligomycin: 12.6 μM, FCCP: 20 μM and antimycin: 20 μM) were prepared in aCSF assay medium and preloaded into reagent delivery chambers for automated injections to the tissue at given time points. Oxygen consumption rate of SCs Cells (8 × 10 4 ) were seeded into PLL-pre-coated XF24 plates. After 24 h, the cells were washed two times with PBS and the media were changed to XF Assay medium (modified DMEM from Seahorse Bioscience), containing 2.5 M glucose and 100 mM pyruvate, 30 min before starting the experiment and incubated at 37 °C in CO 2 -free incubator to allow temperature and pH equilibration and loaded into the XF analyzer machine. Concentrations of drugs used on cells were: oligomycin: 1 μM, FCCP: 3 μM and antimycin: 10 μM. Lactate and citrate assay Extracellular lactate and citrate were measured from culture supernatants using lactate and citrate assay kits following manufacturer’s instructions (Biovision, Milpitas, CA). CS activity assay CS activity was measured using Biovision kit (Biovision) following manufacturer’s instructions and results were normalized with protein concentration in each sample. Glucose measurement Glucose concentration in the culture supernatants was measured using Accu-Chek Aviva Glucometer (Roche Diagnostics, Indianapolis, IN) following manufacturer’s instructions. Trimethylrhodamine methyl ester staining SCs (10 × 10 4 ) were seeded into 24-well plates. After 24 h, cells were treated with 20 μM trimethylrhodamine methyl ester for 30–45 min at RT in dark. At least 100 images of each of control and Lkb1 -mutant SCs were taken and fluorescence measurements were done using the Image J software V1.47F. Locomotion and behaviour tests These tests were done and animals were scored as described before [59] . All experiments were done during the light cycle. Multiple behaviour tests were done on different days on the same groups of animals. Mass spectrometry-based lipidomics Extraction of lipids from mouse nerve tissues . Sciatic nerves were weighed and homogenized for 1 min (Tissue Trearor, Biospec Products) in a mixture of water (0.7 ml) and methanol:chloroform (2:1, v/v, 3 ml) after addition of a cocktail of internal standards including [ 2 H 7 ]cholesterol, C12-glucosylceramide (GC), C12-galatosylceramide, D31-PC, C12-sulphatide and C17-ceramide (Cer). The procedure was repeated with methanol (1 ml) in another glass tube to ensure complete recovery of the tissue sample. After sonication of the whole homogenate for 20 min, the solution was centrifuged (3 min at 4,000 r.p.m.) and supernatants transferred to glass tubes. Samples were extracted second round with a mixture of organic solvents of chloroform:methanol:isopropanol:hexane (2:1:1:1, v/v). Samples were filtered through glass wool to recover filtrate. The combined extracts were dried under a stream of nitrogen gas. Different reconstitution solutions were used for different lipid analysis before injection. Preparation of standards and samples for LC–MS/MS analysis . Stock solutions of lipid standards (1 mg ml −1 ) were prepared in chloroform:methanol (1:4, v/v) and stored at −20 °C. Working solutions were prepared by dilution of the stock solutions with methanol. Calibration curves were constructed for cholesterol, PC, Cer, GC and sulphatide standards with internal standard of each class of compounds as in samples. Quantification of Cer, GC, PC and sulphatide with various chain lengths was accomplished using the curve for the compound of the closest structure. The biological extract was reconstituted with different solvents (200 μl) and 10 μl was injected on column for liquid chromatography–tandem mass spectrometry (LC–MS/MS) analysis. Analysis was carried out by LC–electrospray ionization–MS/MS (LC–ESI–MS/MS) using a Waters Quattro Micro API triple quadrupole mass spectrometer (Milford, MA) interfaced with Acquity UPLC system. Nitrogen was the nebulizer gas and argon was the collision gas. The source temperature was maintained at 120 °C, and the desolvation temperature was maintained at 425 °C. The drying gas (N 2 ) was maintained at ca. 800 l per hour and the cone flow gas was turned off. The multiplier was set at an absolute value of 650 V. Optimized parameters, that is, cone voltage and collision energy for cholesterol, GC, Cer, sulphatide and PC were determined by prior infusion of the individual compounds. For quantification of these species, the ESI–MS/MS was operated in the multiple reaction monitoring mode. Online chromatographic separation of subspecies within each class of lipid was achieved using four different LC solvent systems and conditions. Statistical analysis . Paired and unpaired two-tailed student’s t -test was used to calculate statistical significance, with P <0.05 representing a statistically significant difference. How to cite this article: Pooya, S. et al. The tumour suppressor LKB1 regulates myelination through mitochondrial metabolism. Nat. Commun. 5:4993 doi: 10.1038/ncomms5993 (2014).